Competitive and cooperative metabolic interactions in bacterial communities Revealing the ecological principles that shape communities is a major challenge of the post-genomic era. To date, a systematic approach for describing inter-species interactions has been lacking. Here we independently predict the competitive and cooperative potential between 6,903 bacterial pairs derived from a collection of 118 species' metabolic models. We chart an intricate association between competition and cooperation indicating that the cooperative potential is maximized at moderate levels of resource overlap. Utilizing ecological data from 2,801 samples, we explore the associations between bacterial interactions and coexistence patterns. The high level of competition observed between species with mutual-exclusive distribution patterns supports the role of competition in community assembly. Cooperative interactions are typically unidirectional with no obvious benefit to the giver. However, within their natural communities, bacteria typically form close cooperative loops resulting in indirect benefit to all species involved. These findings are important for the future design of consortia optimized towards bioremediation and bio-production applications. A fundamental question in ecology is how different species can coexist in nature. Darwin's famous documentation of the nutritional divergence within a family of finches resulted in the principle of competitive exclusion, which asserts that coexistence is made possible through divergence and the subsequent reduction in resource overlap (RO) [1] , [2] . However, the observed phenotypic similarity between co-occurring species has led to renewed questioning about the role of competitive interactions in shaping communities; it has been suggested that the carrying capacity of many environments is sufficient to allow the coexistence of closely related species [3] . In addition to competition, growing evidence supports the prevalence of cooperative interactions between organisms [4] , [5] , [6] , [7] . Yet, despite their prevalence, the consequences of cooperative interactions for species diversity are yet poorly understood [8] . The analysis of species' co-occurrence data has long been used by ecologists to discern the forces that dictate community structure [9] , [10] . Yet, to date, empirical records of species' distribution have been highly fragmented, and a systematic approach for estimating the corresponding levels of inter-species competitive and cooperative interactions has been lacking. Within bacterial communities, competitive (where two species consume shared resources) and cooperative (where the metabolites produced by one species are consumed by another and, potentially, vice versa) interactions are to a large extent derived from metabolism. Stoichiometry-based metabolic models were recently shown to provide accurate predictions for the patterns of metabolic interactions in bacterial two-species systems [11] , [12] , [13] , making these approaches a useful tool for exploring ecological concepts [7] . Beyond focusing on a few well-defined case studies, stochiometric constraint-based modelling (CBM) was already used for the systematic design of cooperation-supporting media for all pair-wise combinations formed between seven microorganisms represented by genome-scale metabolic models [13] . Yet, the relative scarcity of such manually curated models has precluded the conductance of larger-scale explorations. Moreover, the ecological significance of these interactions has not been examined on a large scale. Very recently, an automatic high-throughput reconstruction pipeline has generated >100 genome-scale metabolic bacterial models spanning 13 bacterial divisions [14] . This development, complemented by the recent accumulation of metagenomics data from environmental surveys, has now provided a golden opportunity to perform systematic inter-species in silico studies on an ecological scale. Previous large-scale computational studies of microbial ecology and metabolism relied solely on network representations of enzymes and reactions [15] , [16] , [17] (rather than representation by an operative stoichiometry-based metabolic model), and such studies lacked the tools for systematically describing pair-wise interactions in a media-dependent manner. Here, we present the results of the first integrative computational and ecological study that aims to provide a global-scale description of bacterial metabolic interactions between geographically co-occurring, mutually exclusive and randomly distributed species pairs. To this end, we define a conceptual computational framework for characterizing the levels of metabolic competitive and cooperative interactions between pairs of species. Subsequently, we explore the distribution patterns of species as derived from environmental samples in order to relate their ecological co-occurrences to the types of interactions inferred. In silico and in vivo description of co-growth patterns Starting from a collection of 118 genome-scale metabolic models of bacteria, we systematically used CBM for computing the biomass production rate for each of the individual species and their corresponding 6,903 pair-wise combinations (Methods). Analogously to the computation of genetic interactions [18] , we assume three types of potential interactions ( Fig. 1 ): negative, where two species consume shared resources (competition); positive, where the metabolites produced by one species are consumed by another; and potentially vice versa (representing mutualism, commensalism or parasitism—that is positive/positive, positive/neutral or positive/negative interactions), hence producing a synergic co-growth benefit; and neutral, where co-growth has no net effect ( Fig. 1 ). As in genetic interactions, the extent and type of interactions occurring between two species can be described by comparing the total biomass production rate in the pair-wise system to the sum of the corresponding individual rates recorded in their individual growth. 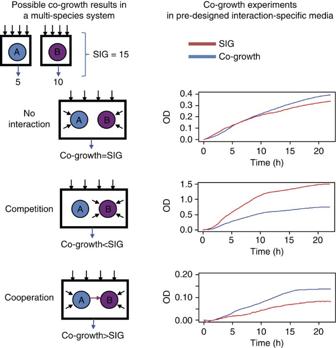Figure 1: Metabolic modelling in a multi-species system. The scheme on the left is an illustrative example of potential interaction types occurring between species in a pair-wise system. No interaction is expected when species A and species B use non-overlapping resources of the corresponding environment; negative interaction/competition: decrease in the overall growth is expected when species A and species B share the same resources; positive interaction/cooperation: increase in the overall growth is expected when the products of one species are the substrates of the second species. On the right: co-growth experiments ofL. innocuaandA. tumefaciensin three interaction-specific (no interaction, competition and cooperation), computationally pre-designed media. Species were grown in a defined medium modified forListeriagrowth. Computational predictions for the experiments: no interactions: SIG(83.1)=∼CG(87.5); competition: SIG(109.2)>CG(97.3); cooperation: SIG(0.0) Figure 1: Metabolic modelling in a multi-species system. The scheme on the left is an illustrative example of potential interaction types occurring between species in a pair-wise system. No interaction is expected when species A and species B use non-overlapping resources of the corresponding environment; negative interaction/competition: decrease in the overall growth is expected when species A and species B share the same resources; positive interaction/cooperation: increase in the overall growth is expected when the products of one species are the substrates of the second species. On the right: co-growth experiments of L. innocua and A. tumefaciens in three interaction-specific (no interaction, competition and cooperation), computationally pre-designed media. Species were grown in a defined medium modified for Listeria growth. Computational predictions for the experiments: no interactions: SIG(83.1)= ∼ CG(87.5); competition: SIG(109.2)>CG(97.3); cooperation: SIG(0.0) Full size image Naturally, interactions between a pair of species are expected to vary significantly depending on the given growth environment. Consequently, for a given pair of species, we can design different media that may reveal different types of interactions. The predictive power of our simulation in inducing shifts from neutral to negative and positive interactions was experimentally tested for 10 bacterial pairs, representing all possible pair-wise combinations between five species capable of growing in the same defined media (IMM, Methods). For all combinations, we simulated co-growth in the original defined media as well as in a range of modified media formed by the addition and subtraction of specific nutrient combinations, leading to the selection of two-media compositions that induce maximal negative and positive shifts, respectively (Methods). Laboratory co-growth experiments were then conducted for all species pairs across the three designed media (original, negative and positive) where positive and negative shifts were correctly predicted in 65% of the experiments (precision 0.75, recall 0.8, Supplementary Note 1 ). The observed and predicted interactions between Listeria innocua and Agrobacterium tumefaciens , demonstrating a close to neutral interaction in the original defined media, are shown in Figure 1 . As evident, shifts from neutral to negative and positive interactions between the two species are successfully induced in the designed media, testifying to the model's predictive ability. Notably, one should bear in mind that our experiments only cover a small subset of all potential pair-wise interactions. Yet, our experiments join to a growing number of studies testifying for the ability of metabolic-driven computational approaches to describe the metabolic interaction between two species [11] , [12] , [13] , [19] . Systematic predictions of the competitive potential As interactions are condition specific, and because nutrient concentrations in specific natural niches are mostly unknown and subject to significant variations, we subsequently aimed to design simulated media that, for each given pair of species, can efficiently uncover their potential capacity to compete or cooperate. To design a medium that maximizes potential competitive interactions, we followed the traditional perception of competition as a situation with a high level of resource requirement overlap, which precludes resource sharing [20] , [21] , [22] . This approach yielded 6,903 pair-specific in silico minimal optimal media, termed competition-inducing media (COMPM, Methods). For each pair, COMPM includes the minimal set of metabolites, provided at their minimal quantity, yet still allowing each species to individually grow at its maximal possible growth yield, leading to the full consumption of external resources (Methods). Thus, when resources overlap, this medium will uncover potential competition. For each pair of species placed in its respective competition-inducing medium, we predicted the win–lose relationships by comparing the individual biomass production (growth yield) rates within the pair-wise system. Winners (faster species in the pair-wise system) tend to be species with higher potential biomass production rates (the latter determined in a single-species system, Fig. 2a ), in accordance with the notion that faster species out-grow their competitors [23] . Looking at the identity of the frequent winners in silico , we observe a clear correspondence between our predictions and ecological data, where winners include fast growing, ecologically versatile species such as Escherichia coli , Salmonella typhimurium , Vibrio cholerae and Pseudomonas aeruginosa (in accordance with earlier observations [17] ; see Supplementary Note 2 ). Similarly, in silico losers include slow growing specialists such as Mycoplasma genitalium and Buchnera aphidicola . The identification of winners as species with higher individual growth rates is also maintained when considering the experimentally recorded doubling times ( Fig. 2b ). 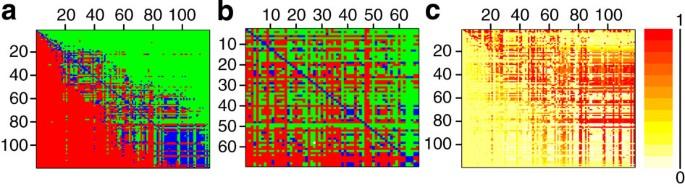Figure 2: Metabolic modelling of pair-wise growth on a COMPM. The matrices describe the outcome of competition between all species pairs. Rows and columns represent species (sorted differently in each slot), where each cell shows the win/lose outcome of the column species following co-growth with the row species. (a,b) Green, red and blue represent win/lose/inconclusive outcome predictions, respectively. Briefly, the winner is defined as the species with the higher predicted growth in a two-species system. (a) Species in rows and columns are sorted according to their computed biomass production rates. Winner–loser relationships were determined for >90% of the pair combinations. (b) Species in rows and columns are sorted according to their experimentally measured doubling times. The predicted win–lose division inbis found to be significantly more distinct than in permuted matrices (Pvalue 0.002). (c) The ratio of biomass production rate of each species in the pair-wise system relatively to its biomass production rate when grown alone. Cells are sorted as in (a). In correspondence with the ecological observation that the faster growing species are the ones exploiting the shared resources [23] , Figure 2c shows that the in silico faster species tend to grow closer to their full capacity than the slow growers (see Supplementary Table S2 for full list of species including the computed and measured doubling times. Computed growth rates of each species across all pair-wise combinations are provided in Supplementary Data 7 ). Figure 2: Metabolic modelling of pair-wise growth on a COMPM. The matrices describe the outcome of competition between all species pairs. Rows and columns represent species (sorted differently in each slot), where each cell shows the win/lose outcome of the column species following co-growth with the row species. ( a , b ) Green, red and blue represent win/lose/inconclusive outcome predictions, respectively. Briefly, the winner is defined as the species with the higher predicted growth in a two-species system. ( a ) Species in rows and columns are sorted according to their computed biomass production rates. Winner–loser relationships were determined for >90% of the pair combinations. ( b ) Species in rows and columns are sorted according to their experimentally measured doubling times. The predicted win–lose division in b is found to be significantly more distinct than in permuted matrices ( P value 0.002). ( c ) The ratio of biomass production rate of each species in the pair-wise system relatively to its biomass production rate when grown alone. Cells are sorted as in ( a ). Full size image Going beyond win–lose predictions, we designed a Potential Competition Score (PCMS, Methods) to quantify the level of competition predicted among the species in our collection, by comparing their individual and combined biomass production rates across simulated COMPM. A PCMS value of 0 denotes no competition and PCMS of 1 indicates maximal competition, while negative PCMS values denote cooperation and synergic co-growth. In all, 98% of the PCMS values are positive (competitive) with a mean PCMS of 0.77 ( Fig. 3a ). As expected, we observe that PCMS values strongly correlate with the degree of in silico RO, the latter determined by the level of intersection between the minimal media sufficient for maximal growth rate of the two species ( Fig. 3b and Methods). 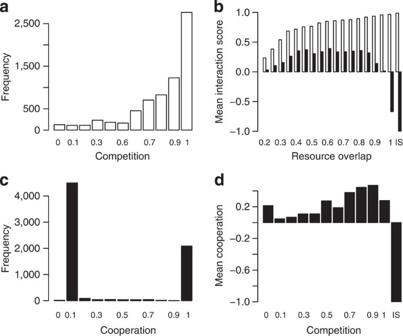Figure 3: Distribution of competition and cooperation values. (a) The distribution of predicted PCMSs across the 6,903 non-redundant species' pairs grown in competition-inducing environments (COMPM). (b) The relation between RO and competition (white) and cooperation (black) scores. RO and competition: Spearman rank correlation 0.4,P-value <2.2e−16. RO and cooperation: correlation coefficient for a second-order polynomial regression 0.3,P-value <2.2e−16. IS (the extreme right bars) indicates intra-species interaction (competition and cooperation values recorded when a species is paired with itself). (c) The distribution of predicted PCPS across the 6,903 non-redundant species pairs grown in COOPM. (d) The relation between cooperation and competition levels: The Spearman correlation between competition and cooperation is significant but very low (0.04,P-value 8e−4). When limiting to intermediate competition values of 0.1<PCMS<0.8, this correlation is more substantial but still quite moderate (0.2,P-value <2.2e−16). Figure 3: Distribution of competition and cooperation values. ( a ) The distribution of predicted PCMSs across the 6,903 non-redundant species' pairs grown in competition-inducing environments (COMPM). ( b ) The relation between RO and competition (white) and cooperation (black) scores. RO and competition: Spearman rank correlation 0.4, P -value <2.2e−16. RO and cooperation: correlation coefficient for a second-order polynomial regression 0.3, P -value <2.2e−16. IS (the extreme right bars) indicates intra-species interaction (competition and cooperation values recorded when a species is paired with itself). ( c ) The distribution of predicted PCPS across the 6,903 non-redundant species pairs grown in COOPM. ( d ) The relation between cooperation and competition levels: The Spearman correlation between competition and cooperation is significant but very low (0.04, P -value 8e−4). When limiting to intermediate competition values of 0.1<PCMS<0.8, this correlation is more substantial but still quite moderate (0.2, P -value <2.2e−16). Full size image Systematic predictions of the cooperative potential Owing to the rich nature of the COMPM, which is likely to conceal inter-species metabolite transfer and cooperation [12] , only very few positive interactions (negative PCMS values) are revealed ( Fig. 3a ). For example, the documented cooperative interaction between the two halophylic species Salinibacter ruber and Haloquadratum walsbyi [24] is only revealed in our simulation setting when reducing their in silico growth medium, inducing the reported dependence of H. walsbyi in S. ruber for the supply of dihydroxyacetone ( Supplementary Note 3 ). We thus computed for each pair of species an in silico minimal medium designed to support a predetermined small level of growth of both species together, termed a cooperation-inducing medium (COOPM, Methods), taking a similar approach as in ref. 13 . Potential Cooperation Scores (PCPS) are then computed according to the ratio between the sum of individual growth rates and the co-growth rate, where positive values indicate cooperation and negative values indicate competition (Methods). Whereas in rich in silico media almost none of the pairs exhibit positive interactions (negative PCMS), about 35% of the pairs show a cooperative potential (positive PCPS) in the in silico COOPM (with scores >0.05, Fig. 3c ). Unlike the monotonic association between similarity in media requirements and the competitive potential described above ( Fig. 3b ), RO and cooperative potential demonstrate an inverted-U relationships ( Fig. 3b ), where a moderate level of similarity in the required resources maximizes the potential for collaboration, and the cooperative potential declines at higher levels of RO. This is likely to stem from the increasing competition on available resources, combined with the scarcity of differing resources that can be shared. Typically, COOPM lack amino acids ( Supplementary Note 4 ), enhancing the need to exchange these metabolites, which were suggested to be transferred between species in mutualistic interactions by ref. 12 . We observe a moderate association between competition and cooperation for intermediate levels of competition ( Fig. 3d ). Interestingly, an inverted-U relationship between RO and cooperation has been reported in economical models describing the likelihood of forming inter-firm alliance versus the corresponding degree of technological overlap. As suggested here for bacterial communities, such economical models suggest that although some degree of technological overlap is necessary to support a successful alliance, at some point such overlap yields diminishing and perhaps even negative returns [25] . Notably, a cooperative potential denotes an overall gain at the pair-wise, system level, though at the species level we can observe a benefit either for both species (mutualism) or to only one of them. Examining the gain of each species in a pair-wise system, we observe that the large majority of in silico cooperative interactions are unidirectional, that is, there is a single species that benefits from the interaction, where the other species is not affected (commensalism, Methods). Similar results were obtained when using alternative approaches for modelling cooperation ( Supplementary Note 5 ). This is in agreement with a recent investigation of computationally predicted pair-wise interactions between seven microbial species across a wide range of environments [13] , and to numerous experimental observations of syntrophic interactions [4] , [24] , [26] , [27] . As displayed in Supplementary Table S1 , one can observe a high tendency of Clostridia species to be involved in cooperative interactions as the giving side. Indeed, Clostridia are known to be involved in the fermentative digestion of cellulose and lignin leading to the subsequent release of easily degradable carbohydrates to other community members [28] , [29] . Patterns of interactions across ecological samples As the benefits to the giver in predicted unidirectional cooperative interactions are not obvious, their relevance for species' coexistence may be questioned. To directly relate the computational predictions to patterns of species coexistence, we used 16S data from environmental surveys across 2,801 samples belonging to 59 different ecological niches [30] . We defined two categories of ecologically associated pairs: pair members that show a similar distribution pattern across the 59 ecological categories are termed niche-associated (648 pairs versus 2,512 non-niche-associated pairs); some of the niche-associated pair members further show a similar distribution pattern across the 2,801 individual samples composing the different ecological categories (niches), and are termed co-occurring pairs (84 pairs, Methods). Competition scores recorded for ecologically associated, and in particular co-occurring, species are significantly higher than those of non-associated pair members ( Fig. 4a ). This is in agreement with the dominant ecological perception of high level of competition between neighbouring species making use of the same resources [3] , [30] . We also observe a significantly higher rate of cooperative give–take interactions between ecologically associated (at both niche and sample level) versus non-associated species ( Fig. 4b ). This observation is retained when compared at different levels of competition and RO ( Supplementary Fig. S1 ), in line with existing ecological theory [8] . 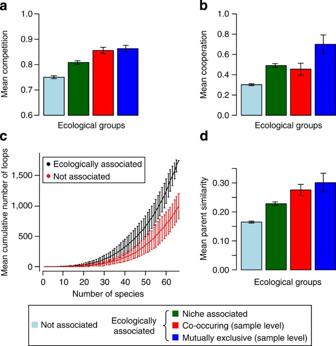Figure 4: Predicted competitive and cooperative interactions across different ecological groups. The level of predicted interaction potential was calculated across randomly distributed and ecologically associated species pairs. Three categories of ecological associations were considered: association at the level of ecological niche, association at the level of the sample (co-occurring pairs) and an antagonistic pattern of distribution at the sample level (mutual-exclusive pairs). (a) Competition scores. (b) Cooperation scores. The difference between ecologically associated and non-associated groups for both competition and cooperation is highly significant (P-value <2.2 e−16, one-sided Kolmogorov–Smirnov test). (c) The mean cumulative number of loops across 1,000 reconstructions of the networks versus the number of species in a network of give–take interactions, for networks of ecologically associated versus networks of non-associated species (Methods). Bars represent standard deviations. (d) Parent similarity, calculated as the fraction of common givers. Bars (ina,bandd) represent standard error. Figure 4: Predicted competitive and cooperative interactions across different ecological groups. The level of predicted interaction potential was calculated across randomly distributed and ecologically associated species pairs. Three categories of ecological associations were considered: association at the level of ecological niche, association at the level of the sample (co-occurring pairs) and an antagonistic pattern of distribution at the sample level (mutual-exclusive pairs). ( a ) Competition scores. ( b ) Cooperation scores. The difference between ecologically associated and non-associated groups for both competition and cooperation is highly significant ( P -value <2.2 e−16, one-sided Kolmogorov–Smirnov test). ( c ) The mean cumulative number of loops across 1,000 reconstructions of the networks versus the number of species in a network of give–take interactions, for networks of ecologically associated versus networks of non-associated species (Methods). Bars represent standard deviations. ( d ) Parent similarity, calculated as the fraction of common givers. Bars (in a , b and d ) represent standard error. Full size image Although the accumulation of some end-product metabolites can be toxic, the advantages for giver species remain obscure. To explore the role of cooperative interactions at the level of the community, we constructed the inter-species network of predicted directional (give–take) interactions (Methods); within this network, we identified motifs of closed cooperative loops, for example, A gives to B; B gives to C; C gives to A (Methods). The occurrence of these closed cooperative loops across natural communities (the 2,801 samples described above) was compared with their occurrence across randomly generated communities preserving the original size and rank of species' distribution. Remarkably, the frequency of loops predicted in natural communities (194) is an order of magnitude higher than in randomly drawn samples (maximum 95 in 1,000 random data sets, mean 10, Supplementary Methods ). Thus, cooperative interactions in nature are likely to be beneficial, forming cooperative cycles. Furthermore, there is a rapid increase in the number of cooperative loops as more species are added in, in particular for ecologically associated species ( Fig. 4c ). This may suggest an explanation to the observed rise in the population size when the species' diversity increases [8] , [31] . A closer examination of the cooperative loops found in natural communities sheds light on how cooperation and competition are intricately intertwined: an illustrative case is that of Pseudomonas putida and Nocardia farcinica , each forming an analogous loop with Streptomyces coelicolor and Bacillus anthracis in two distinct natural samples. As can be expected from their equivalent location inside the loop, the literature suggests that P. putida exhibits a similar role to Nocardia species in the degradation of oil contamination, where the synthetic introduction of P. putida suppresses the enrichment of indigenous degraders such as Nocardia species [32] . To systematically explore the consequences of analogous network positioning for species coexistence, we defined a third group of ecologically associated pairs: mutually exclusive species, referring to pairs of species whose level of coexistence across samples is lower than expected by chance despite the fact they inhabit similar niches (28 pairs, Methods). Figure 4 reveals some interesting trends: we observe that mutually exclusive pairs exhibit high similarity in their network positioning (competing for common givers, Fig. 4d ) as well as high levels of resource competition ( Fig. 4a ), providing systematic evidence for the association of exclusion and competition [1] . Notably, co-occurrence and mutual-exclusion relations may be interchangeable, and the choice between these contradictory fates is determined by the carrying capacity of their environment [3] . Accordingly, similar levels of competition are observed between mutually exclusive and co-occurring pairs ( Fig. 4a,d ). Strikingly, the highest level of cooperative interactions is recorded between mutually exclusive pairs ( Fig. 4b , and Supplementary Note 5 ). This may suggest that under true, natural conditions, cooperative potential, describing the propensity of a species pair to be involved in a unidirectional give–take interaction, might be obscured by competition even to the level of exclusion of one of the pair members. Such is the case with P. putida and Acinetobacter sp. , two highly competing species, which were also predicted to have cooperative potential; when these species were grown experimentally in a deprived environment with benzyl alcohol as the sole carbon source, the benzoate excreted by Acinetobacter sp. was used by P. putida , which subsequently suppressed the growth of Acinetobacter [33] . To date, it has been difficult to predict which bacteria can stably coexist, let alone cooperate metabolically, making the artificial design of beneficial microbial consortia extremely difficult. Here, we suggest a generic approach for the systematic description of inter-species interactions, making use of recently available data. Our approach is obviously not without limitations. First, it is solely aimed at the metabolic dimension while putting aside regulation as well as the numerous strategies that microorganisms have evolved to augment the acquisition of resources. Antimicrobial production, motility and predation can tip the competitive balance, resulting in outcomes that significantly differ from those predicted by simulations restricted to passive nutrient consumption [7] . Moreover, several mechanisms for nutrient sequestration function directly to actively restrict or remove a nutrient from one organism and supply it to another [34] . Second, the analysis lacks information on the true metabolic composition of the environments considered and hence focuses on predicting the overall potential inter-species interactions, rather than providing a direct account of their actual in-vivo communications in one specific environment. Finally, although the automatic reconstruction procedure results in a significant increase in the number of genome-scale metabolic models and although such models have been proven useful in the prediction of a variety of phenotypes, yet they are typically less accurate than manually curated models [14] . Yet, despite these significant limitations, our generic approach succeeds in delineating clear differences in the interaction patterns of ecologically associated and randomly distributed species, pointing at fundamental ecological principles in a systematic fashion. With the increasing efforts to provide an a-biotic description of different environments, together with the expected rapid rise in the number of metabolic models as well as the improvement in their quality, the utilization of metabolic modelling for community-level modelling framework such as the one laid down here provides a computational basis for many exciting future applications. These include the artificial design of 'expert' communities for bioremediation, where currently the selection of community species is done by intelligent guesswork. Similarly, our work may be applied to the rational design of probiotic administration, as well as to the identification of species that may metabolically out-compete pathogenic species. The ability to design and test novel interactions, and to study existing ones means that microbial experiments can be used to complement and extend classical plant and animal ecology, in which many of the principles of biological interactions were first described [27] . Metabolic simulations A total of 118 operative metabolic models were retrieved from The Seed's metabolic models section ( http://seed-viewer.theseed.org/seedviewer.cgi?page=ModelViewer ) [14] . The models are automatically constructed by a pipeline that starts with a complete genome sequence as an input and integrates numerous technologies such as genome annotation, reaction network annotation and assembly, determination of reaction reversibility and model optimization to fit experimental data. The list of species and their corresponding identifiers in the SEED database is provided in Supplementary Table S2 . Briefly, in these models, a stoichiometric matrix ( S ) is used to encode the information about the topology and mass balance in a metabolic network, including the complete set of enzymatic and transport reactions in the system and its biomass reaction. Our approach for generating multi-species models follows the definition employed by ref. 11 . We converted the model of each organism into a compartment in a multi-species system. Applying the multi-species system analysis to all possible pair-wise combinations, we examined 6,903 unique pairs whose growth can be simulated under a range of environments. For a single-species model A, the competition-inducing medium (COMPM) is defined as the ranges of fluxes of the exchange reactions that supports its maximal biomass rate (MBR), when all exchange metabolites are provided at the minimal required amount. For the multi-species system of A and B, COMPM AB allows A and B to reach their MBR at individual growth. However, at co-growth, any RO will prevent species A and B from simultaneously reaching their MBR, and reveal potential sources of competition. A COOPM for a multi-species system is defined as a set of metabolites that allows the system to obtain a small positive growth rate (above a certain predetermined threshold, which may yet be far from optimal), and such that the removal of any metabolite from the set would force the system to have no such solution. A feasible solution in this context is defined as one achieving at least 10% of the joint MBR obtained when grown on a rich medium (COMPM). The processes of models retrieval, calculation of maximal biomass production rate (MBR), construction of pair-wise systems and computation of pair-specific environments (COMPM and COOPM) are fully described in the Supplementary Methods (see also Supplementary Tables S4-S11 and Supplementary Data 8 , 9 , 10 , 11 ). To relate the computed environments to real ecological conditions, we verified that species inhabiting similar environments tend to have similar metabolic profiles, as previously demonstrated in ref. 30 . As documented in many laboratory experiments, typical limiting factors in COMPM environments include oxygen, glucose and nitrogen sources ( Supplementary Note 4 ). Finally, computational simulation providing predictions for the effect of removal of chosen metabolites on species growth were experimentally tested, supporting the ability of the models to identify growth-limiting factors ( Supplementary Note 6 ). Experimental and computational co-growth analysis Co-growth experiments were conducted between all co-growth combinations formed between five species, all non-pathogenic and capable of growing in IMM. The species and their seed models are the following: L. innocua Clip11262 (Core272626_1), A. tumefaciens str. C58 (Core176299_3), E. coli K12 (Core83333_1), P. aeruginosa PAO1 (Core208964_1) and Bacillus subtilis str. 168 (Opt224308_1). Exprimental procedure and media selection are fully described in the Supplementary Methods section. Determining win–lose and give–take relationships In a multi-species system, the CBM solver aims to maximize the total growth potential of all species, and provides a range of potential solutions for the contribution of each compartment to the total growth. We define: where V BM, m is the maximal biomass production rate in a system m , corresponding to species A and B. We define A as a winner when the lowest value of its predicted maximal growth is higher than the highest value predicted for species B. Where V min, BM, COMPM, compartment_A and V max, BM, COMPM, compartment_B (maximal biomass production rate of organism A and B, respectively, in the multi-species system) are calculated when running flux variability analysis (FVA) for the multi-species system and fixating the V BM, AB to its maximal value on the given media. To determine give–take relationships in a multi-species system of species A and B, we look at the individual benefit of each species/compartment when the species are grown together. We define A as a 'Taker' if its maximal growth in the multi-species system is higher than its individual maximal growth in a minimal medium. In this case, we call B a 'Giver' It is of course possible within the same system that species A and B are both 'givers' and 'takers' (a symmetrical interaction). Overall, we observe that 94% of the interactions are unidirectional (commensalism) ( Supplementary Note 5 ). None of the unidirectional interactions affects the growth of the giver (neutral interactions). The directional network of give–take interactions is provided in Supplementary Data 1 . Within this network, we looked for close cooperative loops (that is, A→B, B→C, C→A) up to a size of four species. Determining the level of competition and cooperation PCMSs are calculated as: PCPS are calculated as: where V BM,x,y is the flux through the biomass reaction of species y in medium x. Computed PCMS and PCPS values are provided in Supplementary Data 2 and 3 , respectively. Calculating the RO within a species pair The RO between a pair of species is calculated as the ratio between the intersection and union sizes (Jaccard index) of the set of uptake reactions included in their individual COMPM. Computed RO values are provided in Supplementary Data 4 . Collection of ecological distribution data Data of operational taxonomic units (OTUs) distribution in environmental samples were retrieved from ref. 30 , using their 97% identity threshold for sequence clustering. Each sequence is mapped to a 'sampling event' defined as the unique concatenation of the three annotation fields 'author'+'title'+'isolation_source'. For example, 51 sampling events are mapped to the publication 'Microbial ecology: human gut microbes associated with obesity' [35] . These sampling events refer to 15 different individuals, each under a different diet, at different time points (considering the beginning of the experiment). Notably, in samples from host-associated metagenomic studies, an 'isolation source' is individual specific, as in ref. 35 . 'isolation_source' fields are further mapped to an environment ontology (EnvO) [36] (for example, 'agricultural soil' and 'Rocky Mountain alpine soil' are mapped to the term 'soil'). Overall, 2,662 samples are mapped to 183 EnvO categories, termed 'niches'. As many niches contained only a few samples, we strived to group similar niches together to obtain a better signal. Using the hierarchical clustering in EnvO, we automatically mapped samples from lower order niches to higher order ones. This process continued iteratively until reaching a barrier of predefined niches with no biological significance. Using this approach, the ultimate set contained 59 ecological niches ( Supplementary Table S3 ). Full length 16S rRNA sequences corresponding to the 118 species with metabolic models that were used throughout the analysis were manually retrieved from the Kyoto Encyclopaedia of Genes and Genomes [37] . BLAST [38] was then used to map the models to OTUs, requiring 97% sequence identity and 95% alignment overlap, considering the length of the query sequence. In case of multiple matches for a given OTU, we map it to the model represented by the highest-ranking sequence, thus resulting in a one-to-many mapping between models and OTUs. That is, each OTU can only be mapped to a single model, but a model can be mapped to many OTUs. Overall, 80 models were identified across the environmental samples. Supplementary Data 5 lists the samples tested, their mapping to niches and the detected array of species. Determining ecological association between species To identify ecologically associated species, we examined the distribution pattern of the 80 OTU-mapped models across the 59 niches [36] . The probability that two species co-occur together at a rate higher than chance expectation was determined by calculating a cumulative hypergeometric P- value. Significance cutoff was determined by setting a false discovery rate threshold of 10%. Similarly, we looked at the pattern of species' distribution across the 2,662 samples. We identified 111 non-redundant combinations of co-occurring species and 39 non-redundant combinations of mutually exclusive species from the pairs—that is, species for which the coexistence in samples is higher or lower than expected by chance, respectively. As can be expected, the large majority of co-occurring pairs is observed between ecologically associated species (84/111). Less trivial is the identification of a significant part of the mutually exclusive species pairs (28/39) as ecologically associated species, implying that the pattern of distribution of species in nature is far from being random. Only niche-associated pairs are further analysed as co-occurring (84) or mutually exclusive (28) combinations. The ecological association types determined for the species pairs tested are provided in Supplementary Data 6 . The distribution of RO values between ecologically associated and non-associated pairs is shown at Supplementary Figure S2 demonstrating that ecologically associated pairs differ in the pattern of distribution of their RO values, supporting both the observed high level of competitive and cooperative interactions. The identification of close cooperative loops in real and random networks of give–take integrations and in real and randomly drawn communities is fully described in the Supplementary Methods section. How to cite this article: Freilich, S. et al . Competitive and cooperative metabolic interactions in bacterial communities. Nat. Commun. 2:589 doi: 10.1038/ncomms1597 (2011).